Resolving stepping rotation inThermus thermophilusH+-ATPase/synthase with an essentially drag-free probe Vacuole-type ATPases (V o V 1 ) and F o F 1 ATP synthases couple ATP hydrolysis/synthesis in the soluble V 1 or F 1 portion with proton (or Na + ) flow in the membrane-embedded V o or F o portion through rotation of one common shaft. Here we show at submillisecond resolutions the ATP-driven rotation of isolated V 1 and the whole V o V 1 from Thermus thermophilus , by attaching a 40-nm gold bead for which viscous drag is almost negligible. V 1 made 120° steps, commensurate with the presence of three catalytic sites. Dwells between the steps involved at least two events other than ATP binding, one likely to be ATP hydrolysis. V o V 1 exhibited 12 dwell positions per revolution, consistent with the 12-fold symmetry of the V o rotor in T. thermophilus . Unlike F 1 that undergoes 80°–40° substepping, chemo-mechanical checkpoints in isolated V 1 are all at the ATP-waiting position, and V o adds further bumps through stator–rotor interactions outside and remote from V 1 . The F o F 1 - and V-type ATPase/ATP synthase superfamily utilizes a rotary mechanism to perform their specific functions [1] , [2] , [3] . The basic structures of these ATPases/synthases are conserved among species. The soluble, cytoplasmic portion of F o F 1 - and V-type ATPases (called F 1 and V 1 , respectively), responsible for ATP hydrolysis/synthesis, is connected via the central rotor stalk and the peripheral stator stalk to the transmembrane portion (F o and V o ) that houses the ion-transporting pathway. In the bacterial V-type ATPase of Thermus thermophilus (V o V 1 ), the V 1 portion is composed of a hexameric A 3 B 3 cylinder and a central shaft composed of D and F subunits [4] (see Fig. 1a ). The V o portion of T. thermophilus is composed of two distinct domains: a hydrophobic rotor ring made of V o -c subunits supplemented with a funnel shape V o -d subunit and a stator apparatus composed of a transmembrane V o -a subunit and EG subunits forming the peripheral stalk [5] , [6] (see Fig. 1b ). Cryoelectron micrographs of two-dimensional crystals of the V o ring at 7.0 Å resolution showed the presence of 12 V o -c subunits, each composed of two transmembrane helices [7] . The bacterial V-ATPase that we describe here works as an ATP synthase [1] , whereas its eukaryotic counterpart is vacuolar proton pump and thus some mechanistic differences may exist [1] , [2] , [8] . A number of researchers refer to the bacterial V-ATPase as archaeal-ATPase or A o A 1 -ATP synthase, but here we adopt the broader terminology. 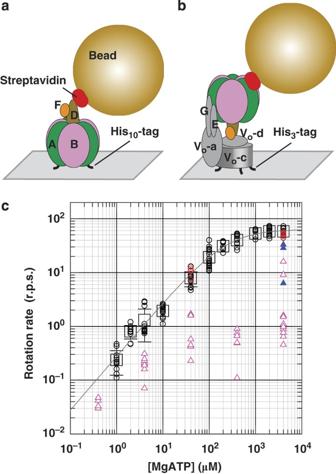Figure 1: Rotation of V1and VoV1carrying a 40-nm bead. Schematic observation systems for rotation of V1(a) and VoV1(b). (a) V1was fixed to the Ni2+-NTA-coated glass surface with his10tags at A subunits. A 40-nm bead (or duplex) was attached to the biotinylated cysteine residues (E48C/Q55C) of the D subunit via streptavidin. In this system, the central shaft composed of D and F subunits rotates relative to A3B3subcomplex containing catalytic sites. (b) VoV1was fixed to the Ni2+-NTA-coated glass surface with His3tags at Vo-c subunits. In this system, the stator apparatus composed of A3B3, E, G and Vo-a subunit rotates relative to the fixed central rotor shaft composed of Vo-c ring, Vo-d, D and F subunits. A 40-nm bead (or duplex) was attached to the AviTag at A subunit(s) by biotin–streptavidin linkage. Bead rotation was observed under an optical microscope with dark-field illumination, and recorded with a high-speed camera at 250–8000 frames per s (fps). (c) Rotation rates of beads attached onto V1(circles) and VoV1(triangles) at the indicated ATP concentrations. Red and black circles indicate in the presence and absence of 0.05% (w/v) DDM, respectively. Squares indcate the averages of V1rotation rates (n≥8; s.d. greater than the symbol size shown with bars). Line indicates the fit with Michaelis–Menten kinetics:V=Vmax·[ATP]/(Km+ [ATP]), whereVmaxandKmare 64 r.p.s. and 229 μM, respectively, giving the apparent ATP-binding ratekonof 0.84×106M−1s−1(3×Vmax/Km). For VoV1, the rotation buffer contained 0.05% DDM. Time-averaged rotation rates of V1or VoV1were estimated over tens of consecutive revolutions as listed inSupplementary Table S1. The molecules of VoV1which showed relatively clean 120° steps are shown as closed blue triangles. Figure 1: Rotation of V 1 and V o V 1 carrying a 40-nm bead. Schematic observation systems for rotation of V 1 ( a ) and V o V 1 ( b ). ( a ) V 1 was fixed to the Ni 2+ -NTA-coated glass surface with his 10 tags at A subunits. A 40-nm bead (or duplex) was attached to the biotinylated cysteine residues (E48C/Q55C) of the D subunit via streptavidin. In this system, the central shaft composed of D and F subunits rotates relative to A 3 B 3 subcomplex containing catalytic sites. ( b ) V o V 1 was fixed to the Ni 2+ -NTA-coated glass surface with His 3 tags at V o -c subunits. In this system, the stator apparatus composed of A 3 B 3 , E, G and V o -a subunit rotates relative to the fixed central rotor shaft composed of V o -c ring, V o -d, D and F subunits. A 40-nm bead (or duplex) was attached to the AviTag at A subunit(s) by biotin–streptavidin linkage. Bead rotation was observed under an optical microscope with dark-field illumination, and recorded with a high-speed camera at 250–8000 frames per s (fps). ( c ) Rotation rates of beads attached onto V 1 (circles) and V o V 1 (triangles) at the indicated ATP concentrations. Red and black circles indicate in the presence and absence of 0.05% (w/v) DDM, respectively. Squares indcate the averages of V 1 rotation rates ( n ≥8; s.d. greater than the symbol size shown with bars). Line indicates the fit with Michaelis–Menten kinetics: V = V max ·[ATP]/( K m + [ATP]), where V max and K m are 64 r.p.s. and 229 μM, respectively, giving the apparent ATP-binding rate k on of 0.84×10 6 M −1 s −1 (3× V max / K m ). For V o V 1 , the rotation buffer contained 0.05% DDM. Time-averaged rotation rates of V 1 or V o V 1 were estimated over tens of consecutive revolutions as listed in Supplementary Table S1 . The molecules of V o V 1 which showed relatively clean 120° steps are shown as closed blue triangles. Full size image It is believed that V o (and F o ) is a rotary motor driven by the transmembrane flow of protons (or Na + ) and V 1 (and F 1 ) is another rotary motor driven by ATP hydrolysis, and that the two motors have a common rotary shaft yet their genuine rotary directions are opposite to each other. Thus, when V o (F o ) takes control, V 1 (F 1 ) is rotated in reverse direction, ending in the synthesis of ATP. Powering V 1 (F 1 ), on the other hand, results in proton pumping [9] . According to a model for V o and F o , a proton enters an access channel and binds to a glutamate on one of the c subunits in the rotor ring and after one revolution of the ring, the proton is released to the other side of the membrane via an exit channel [10] . In this model, the copy number of the c subunit of V o or F o in the rotor ring is equal to the number of transported protons per revolution. For the T. thermophilus V-ATPase, 12 protons are expected per revolution. The ATP-driven rotation of the DF shaft in V 1 has been observed directly [11] : a bead (nominal diameter 0.56 μm) attached to the D subunit rotated unidirectionally anticlockwise when viewed from the membrane side. At low ATP concentrations where ATP binding is rate limiting, the rotation proceeded in steps of 120°, commensurate with the presence of three catalytic sites at A–B interfaces [12] . Rotation of the V o -c ring in V o V 1 has also been observed [13] , with 120° steps at low ATP concentrations [14] . For F 1 , which also undergoes anticlockwise 120° stepping at low ATP, high-speed imaging with 40-nm gold particles, with little drag, has revealed that a 120° step consists of 80–90° and 40–30° substeps [15] . F 1 cycles through an ATP-waiting dwell, ∼ 80° substep rotation driven by ATP binding and subsequent ADP release, a catalytic dwell where ATP is hydrolyzed and the phosphate is released, and ∼ 40° substep rotation driven by the phosphate release [16] . ATP-driven rotation of F o F 1 has also been demonstrated for Escherichia coli and thermophilic Bacillus PS3 enzymes, with features basically similar to those of F 1 [17] , [18] , [19] . So far, ATP-driven rotation either in V o V 1 or in F o F 1 has failed to reveal a sign of specific interactions between a rotor and a stator subunit in the V o /F o portion, even in the high-resolution study [17] . Here, we have analysed ATP-driven rotation of both V 1 and V o V 1 (holo V-ATPase) derived from T. thermophilus , using a 40-nm bead and a submillisecond fast camera. V 1 molecules rotated with 120° steps without adopting the 80°–40° substep scheme of F 1 . V o V 1 , in contrast, showed ∼ 30° steps that likely reflect stator–rotor interactions in the V o domain. All rate-limiting reactions in the V 1 chemo-mechanical cycle occur in one angle, whereas stator–rotor interactions in V o pose additional bumps that might check rotation depending on protonation/deprotonation. Stepwise rotation of V 1 V 1 was immobilized on a nickel-nitrilotriacetic acid (Ni 2+ -NTA )-coated glass surface through His (histidine) 10 -tags introduced at the amino terminus of the A subunits, and a 40-nm streptavidin-coated gold colloid (40-nm bead) was attached to the biotin-labelled D subunit ( Fig. 1a ). Bead rotation was imaged by laser dark-field microscope and recorded on a fast-framing CMOS camera at speeds up to 8,000 frames per s. ATP dependence of the time-averaged rotation rate of V 1 is shown in Figure 1c . Below 100 μM, ATP binding was rate limiting, the rotation speed being practically proportional to the ATP concentration ([ATP]). The rate constant for apparent, or effective, ATP binding was 0.8×10 6 M −1 s −1 , assuming three ATP molecules consumed per revolution. Above 1 mM ATP, the rotary speed saturated, reaching V max of 64 revolutions per s (r.p.s.). This is the full speed of V 1 rotation at 23 °C, not limited by the viscous drag on the bead (see below). The Michaelis–Menten constant, K m , of 229 μM ( Fig. 1c ) agrees with that for the bulk ATP hydrolysis assay without beads of 205 μM [14] , supporting the contention that V max above represents the speed of unloaded rotation (the reported maximal hydrolysis activity of 39.9 s −1 is lower than 180 s −1 expected for rotation at ∼ 60 r.p.s., because of MgADP inhibition [14] , [15] ). Even at saturating [ATP], all 40-nm beads rotated stepwise, pausing every 120° ( Fig. 2a ), reminiscent of the unloaded rotation of F 1 at saturation. The 120° steps were completed within 0.25 ms (two frames), indicating that V 1 can drive the 40-nm bead at >480° ms −1 , and thus mechanical stepping does not limit the overall rotation rate. The average rotation speed of 64 r.p.s. at saturating [ATP] is limited by the ∼ 5 ms dwells where a reaction(s) that does not accompany rotation takes place. The 120° steps at saturating [ATP] were not resolved in the previous study with a 340-nm bead duplex [12] , where the time-averaged rotation speed at saturation was also low, limited by viscous drag on the large beads. 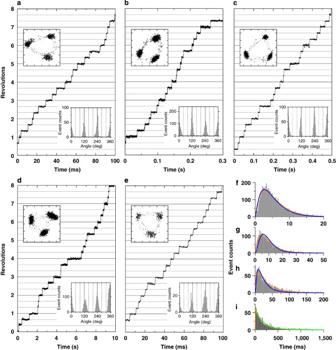Figure 2: Rotation of V1. (a–e) Typical time courses of rotation with a 40-nm bead (or duplex). (a) Rotation at 4 mM ATP captured at 8,000 fps; (b) 200 μM ATP at 2,000 fps; (c) 40 μM ATP at 250 fps; (d) 4 μM ATP at 4,000 fps and (e) 2 mM ATP at 4,000 fps, obtained from the same molecule as indafter medium exchange. Trajectories of the bead centroid (axis divisions: 11.1 nm) and histograms of angular positions, both for the indicated portion of the records, are shown in the upper and lower insets, respectively. (f–i) Histograms of dwell times between 120° steps. (f) Dwell times at 4 mM ATP with 125 μs bin size obtained from 6 molecules observed at 8,000 fps; (g) 200 μM ATP, 250 μs bin size, 6 molecules at 8,000 fps; (h) 40 μM ATP, 1 ms bin size, 6 molecules at 4,000 fps; (i) 4 μM ATP, 4 ms bin, 15 molecules at 2,000 fps. Orange curves show fit with the sequential two-reaction scheme with rateskaandkb: constant·(exp(−kat) − exp(−kbt)). At 4 mM ATP, the two rates turned out to be indistinguishable and thus the fit was made with two identical ratesk: constant·t·exp(−kt). The estimated rates and associated s.e. are:k4 mM=0.36±0.01 ms−1,ka200 μM=0.17±0.02 ms−1,kb200 μM=0.28±0.03 ms−1,ka40 μM=31±1 s−1,kb40 μM=0.40±0.03 ms−1, andka4 μM=6.1±0.1 s−1,kb4 μM=0.26±0.02 ms−1. If we assume thatkarepresents the rate of ATP binding (ka=kon[ATP]),konis given as 0.85×106M−1s−1at 200 μM ATP, 0.78×106M−1s−1at 40 μM and 1.5×106M−1s−1at 4 μM. At 4 μM,konshould dominate the histogram, and the green fit with constant·exp(−kon[ATP]t) gavekonof 1.5×106M−1s−1. Blue curves show a global fit tof–h(equal weight for each count), with sequential reactions starting with ATP binding at the ratekon[ATP] and two ATP-independent reactions with ratesk1andk2: constant·{(k2−k1)·exp(−kon[ATP]t) + (kon[ATP]−k2)·exp(−k1t) + (k1−kon[ATP])·exp(−k2t)} withkon=(1.2±0.1)×106M−1s−1,k1=0.49±0.05 ms−1,k2=0.34±0.04 ms−1. Figure 2: Rotation of V 1 . ( a – e ) Typical time courses of rotation with a 40-nm bead (or duplex). ( a ) Rotation at 4 mM ATP captured at 8,000 fps; ( b ) 200 μM ATP at 2,000 fps; ( c ) 40 μM ATP at 250 fps; ( d ) 4 μM ATP at 4,000 fps and ( e ) 2 mM ATP at 4,000 fps, obtained from the same molecule as in d after medium exchange. Trajectories of the bead centroid (axis divisions: 11.1 nm) and histograms of angular positions, both for the indicated portion of the records, are shown in the upper and lower insets, respectively. ( f – i ) Histograms of dwell times between 120° steps. ( f ) Dwell times at 4 mM ATP with 125 μs bin size obtained from 6 molecules observed at 8,000 fps; ( g ) 200 μM ATP, 250 μs bin size, 6 molecules at 8,000 fps; ( h ) 40 μM ATP, 1 ms bin size, 6 molecules at 4,000 fps; ( i ) 4 μM ATP, 4 ms bin, 15 molecules at 2,000 fps. Orange curves show fit with the sequential two-reaction scheme with rates k a and k b : constant·(exp(− k a t ) − exp(− k b t )). At 4 mM ATP, the two rates turned out to be indistinguishable and thus the fit was made with two identical rates k : constant· t ·exp(− kt ). The estimated rates and associated s.e. are: k 4 mM =0.36±0.01 ms −1 , k a 200 μM =0.17±0.02 ms −1 , k b 200 μM =0.28±0.03 ms −1 , k a 40 μM =31±1 s −1 , k b 40 μM =0.40±0.03 ms −1 , and k a 4 μM =6.1±0.1 s −1 , k b 4 μM =0.26±0.02 ms −1 . If we assume that k a represents the rate of ATP binding ( k a = k on [ATP]), k on is given as 0.85×10 6 M −1 s −1 at 200 μM ATP, 0.78×10 6 M −1 s −1 at 40 μM and 1.5×10 6 M −1 s −1 at 4 μM. At 4 μM, k on should dominate the histogram, and the green fit with constant·exp(− k on [ATP] t ) gave k on of 1.5×10 6 M −1 s −1 . Blue curves show a global fit to f – h (equal weight for each count), with sequential reactions starting with ATP binding at the rate k on [ATP] and two ATP-independent reactions with rates k 1 and k 2 : constant·{( k 2 − k 1 )·exp(− k on [ATP] t ) + ( k on [ATP]− k 2 )·exp(− k 1 t ) + ( k 1 − k on [ATP])·exp(− k 2 t )} with k on =(1.2±0.1)×10 6 M −1 s −1 , k 1 =0.49±0.05 ms −1 , k 2 =0.34±0.04 ms −1 . Full size image At lower [ATP], we still observed 120° steps ( Fig. 2b–d ) without a clear sign of substeps as with F 1 (refs 15 , 16 ). Even at 200 μM ATP, around K m where F 1 would repeat ∼ 80° and ∼ 40° substeps with equal dwells in between, V 1 underwent 120° stepping ( Fig.2b and insets therein). The V 1 dwells at low [ATP] must be at ATP-waiting angles, implicating that the ∼ 5 ms dwells at saturating [ATP] were also at, or close to, ATP-waiting angles. This was also confirmed by solution exchange: Figure 2d,e show rotation of the same V 1 molecule, showing that dwell positions at both high and low [ATP] do not differ significantly. Events that underlie the V 1 dwell V 1 dwells basically (see below) at every 120°, or once per catalytic cycle, irrespective of [ATP]. We now enquire what causes these dwells. At least four events occur in a catalytic cycle of V 1 : ATP binding, ATP hydrolysis, phosphate release and ADP release. Of these, ATP binding must trigger, and likely drives at least partially, the 120° step. Our previous study [12] with a slowly hydrolyzed ATP analogue ATP-γ-S indicated that ATP hydrolysis occurs at an ATP-waiting angle, and thus the time required for hydrolysis is a determinant of the dwell. To see whether hydrolysis alone is responsible for the dwell, we have analysed the distribution of dwell times, measured as the time between the midpoints of two successive 120° steps ( Fig. 2 f–i ). At all four [ATP] examined, the dwell-time histogram was not exponential and rose from the origin (not well resolved at 4 μM), indicating the involvement of two or more rate-limiting reactions. Sequential two-reaction scheme could reasonably fit the histograms (orange lines in Fig. 2f–i ). At 4 mM ATP, the two rates seemed indistinguishable and were 0.36 ms −1 . One rate should correspond to that of ATP hydrolysis, unless a third reaction is also involved. The nature of the other reaction is unknown, but it cannot be ATP binding, which must be rapid at 4 mM ATP (binding rate for ATP is calculated as 3.2 ms −1 by multiplying 4 mM by 0.8×10 6 M −1 s −1 ). Likely candidates are phosphate or ADP release (or both combined). At and below 200 μM ATP, the dwells must also involve the time for ATP binding in addition to the two (or more) reactions at 4 mM. We therefore attempted a global fit to the three histograms ( Fig. 2f–h , blue lines) around K m where the rise from the origin was well resolved, with a sequential scheme for three reactions, of which one is ATP binding with the apparent rate constant k on . Although the fit was not perfect, the recovered k on of 1.2×10 6 M −1 s −1 is consistent with that for 4 μM ATP, and with the estimate from Figure 1c above and a previous value of ∼ 1.3×10 6 M −1 s −1 obtained with 220-nm duplex beads [14] . The other two rates were 0.49 ms −1 and 0.34 ms −1 , roughly consistent with the two-rate fit of the 4 mM dwells above. In addition to the relatively clean 120° steps as in Figure 2 , some beads (52 out of 169; see Supplementary Table S1 ) exhibited peculiar fluctuations such as jumping to and fro between two angles separated by ∼ 40° (see Supplementary Fig. S1 ). Because the basic 120° stepping feature was preserved, we ignore these minor fluctuating beads in the analyses above. Rotation of V o V 1 To examine the effect(s) of the V o domain on the ATP-driven rotation of V 1 in intact V o V 1 , we constructed the experimental system in Figure 1b . V o V 1 was fixed, in the presence of 0.05% (w/v) N-dodecyl β- D -maltoside (DDM) upside down on a Ni 2+ -NTA-coated glass surface via His 3 tags on the V o -c subunits. A 40-nm gold bead was attached to V 1 -A subunit(s) through the Avitag–biotin–streptavidin linkage. Immediately after infusion of millimolar ATP, we found a few rotating beads per field of view (7.1×7.1 μm 2 ). The number decreased with time, particularly at high [ATP] where finding the rotation became difficult after 1 h. Both V o V 1 and V 1 are highly susceptible to ADP inhibition even in the presence of an ATP-regeneration system [14] , [20] . Part of the dormant molecules was somehow reactivated by re-infusion of the observation buffer, allowing further observations. All molecules that rotated for many revolutions (as listed in Supplementary Table S1 ) without an obvious sign of obstruction at a particular angle were subjected to analysis. Rotation speed of V o V 1 was variable and was distributed around 1–10 r.p.s. at 4 mM ATP ( Fig. 1c ). 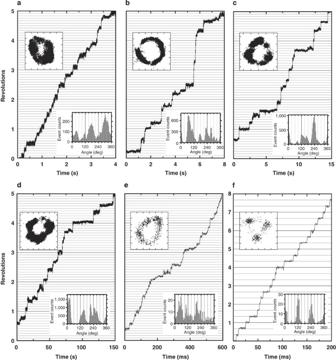Figure 3: Rotation of VoV1. Typical time courses of the rotation of a 40-nm gold bead attached on VoV1in the presence of 0.05% DDM. Horizontal lines are 30° apart, except inf. (a) Rotation at 4 mM ATP captured at 2,000 fps; (b) 40 μM ATP at 2,000 fps; (c) 4 μM ATP at 1,000 fps and (d) 400 nM ATP at 250 fps. (e) A relatively fast rotation (∼10 r.p.s.) with small substeps at 4 mM ATP captured at 1,000 fps. (f) A minor case of rotation with 120° steps at 4 mM ATP captured at 2,000 fps. Trajectories of the bead centroid (axis divisions: 11.1 nm) and histograms of angular positions for the indicated portion of the records are shown in the upper and lower insets, respectively. Typical rotation time courses are shown in Figure 3a–e . Unlike V 1 , which basically paused every 120°, V o V 1 made short pauses at many angles at all [ATP] examined. A relatively fast rotation ( ∼ 10 r.p.s.) at 4 mM ATP is shown in Figure 3e , which still contains many pauses. At this [ATP], most V 1 molecules rotated much faster, at ∼ 60 r.p.s. ( Fig. 1c ). The V o domain seems to introduce bumps that lead to the small steps and the reduced average speed of V o V 1 rotation. In this observation system, the whole stator apparatus (A 3 B 3 EGV o -a) rotates against the central rotor spanning the V o V 1 (DFV o -d V o -c ring). The bumps likely represent the interaction between V o -c ring and V o -a in the V o domain. In 15 analysed molecules, we found three beads that showed clean 120° steps ( Fig. 3f ), and these beads ( Fig. 1c , blue triangles) rotated fast (> ∼ 30 r.p.s.). Detailed analyses of the short pauses in the presence of Triton below suggest that these 120° stepping beads are attached to defective V o V 1 in which the V o interaction is somehow impaired, although the opposite possibility of short pauses being an artefact cannot be ruled out. Figure 3: Rotation of V o V 1 . Typical time courses of the rotation of a 40-nm gold bead attached on V o V 1 in the presence of 0.05% DDM. Horizontal lines are 30° apart, except in f . ( a ) Rotation at 4 mM ATP captured at 2,000 fps; ( b ) 40 μM ATP at 2,000 fps; ( c ) 4 μM ATP at 1,000 fps and ( d ) 400 nM ATP at 250 fps. ( e ) A relatively fast rotation ( ∼ 10 r.p.s.) with small substeps at 4 mM ATP captured at 1,000 fps. ( f ) A minor case of rotation with 120° steps at 4 mM ATP captured at 2,000 fps. Trajectories of the bead centroid (axis divisions: 11.1 nm) and histograms of angular positions for the indicated portion of the records are shown in the upper and lower insets, respectively. Full size image Approximately 30° stepping The detergent Triton X-100 (Triton) has been reported to be deleterious to the integrity of F o F 1 , presumably affecting stator–rotor interaction in F o [21] . Unexpectedly, however, the substep behaviour of V o V 1 above, indicative of rotor–stator interaction in the V o domain, was enhanced when DDM was replaced with Triton. The small substeps could be more clearly discerned in the presence of Triton. When Triton-solubilized V o V 1 was reconstituted into liposomes, it actively pumped protons, indicating that Triton treatment leaves V o V 1 intact [22] . The same lot of V o V 1 has also been shown to be inactivated by N,N′-dicyclohexylcarbodiimide [14] , another sign of integrity particularly in the V o portion. Below, we analyze the clearer substeps observed in the presence of Triton. Somehow, rotation trajectory of V o V 1 was unstable in the presence of a detergent, whether Triton or DDM, and gradually drifted both rotationally and translationally up to a few nanometres. Nevertheless, we could identify pauses clearly in trajectories of successive segments for one to two revolutions ( Fig. 4a , square insets, with frames coloured as in the segmented time course). We could also estimate pausing angles by fitting an ellipse to each segmented trajectory and assuming that the ellipse represents the projection of a circular orbit oblique to the glass surface ( Fig. 4b ). 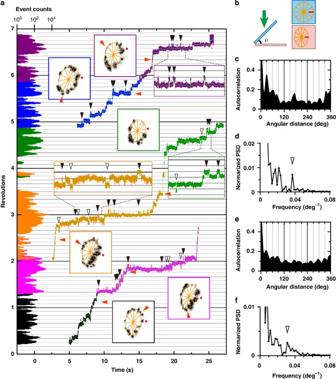Figure 4: Well-resolved substeps in VoV1. (a) An expanded time course of the rotation of a 40-nm gold bead attached on a VoV1at 40 μM ATP, in the presence of 0.1% (w/v) Triton captured at 2,000 fps. Horizontal lines are 30° apart. The time course is split into three and horizontally shifted (magenta and orange curves partially overlap). To minimize the effect of small, gradual drift on the angle analysis, the record was divided into six coloured portions (black, magenta, orange, green, blue and purple) covering∼1 revolution and analysed as follows. First, the bead trajectory in each portion (coloured square insets; grey points show raw data and black after 21-point median filtering ofxandytime courses) was fitted with an ellipsoid (orange). Rotary angle was calculated by assuming the ellipsoid to be a projection of a circular orbit (b). The angle 0, a start of a revolution on the vertical axis of the figure, was assigned to the red dot in each inset, chosen from the 12 orange spokes that fitted the dwells. The green line on the time courses shows 41-point (20 ms) median. The histograms on the left axis represent logarithm of the number of data points per 2°. Red arrowheads, dwells that are clearly out of the 30° periodicity. Black arrowheads, excursions to a neighbouring (closed, forward; open, backward) dwell position for >20° and >20 ms. Boxes enclosing trajectories show a fixed 89×89 nm2area, such that drifts manifest as differences between insets. (b) Circular orbit (cyan) of a bead projected on the image plane (pink). Direction of observation is indicated by a green arrow. For the data ina, the angleθranged between 43° and 55°. (c) The autocorrelation of the angular histogram derived froma; the continuous time course over 2,500° was 21-point median filtered and then binned at 0.25° intervals. For this analysis, we calculated the angular histogram without adjusting the angular origins of the six portions, that is, without correction for the rotational drift, to eliminate possible subjectivity. (d) The power spectrum ofc, the arrowhead showing a peak at (27°)−1. (e) The average of autocorrelations of individual angular histograms forFigures 4c,5candSupplementary Figures S2a,b. (f) The power spectrum ofe, the arrowhead showing a peak at (32°)−1. The angular histogram of the time course is shown on the left axis of Figure 4a . In most parts, the histogram as well as the trajectories show dwells that occur every ∼ 30°, missing positions ascribed to rapid passage. An autocorrelation of the histogram, equivalent with the pairwise angular distribution function [23] , [24] , is shown in Figure 4c together with its power spectrum ( Fig. 4d ). The latter shows a peak at (27°) −1 , indicated by the arrowhead at the resolution of ∼ 4°. 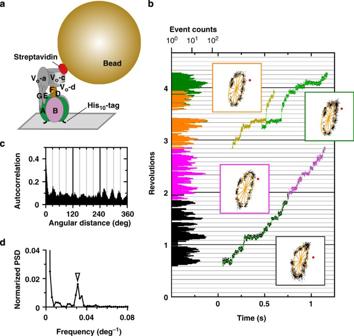Figure 5: Substep rotation in upside up VoV1. (a) Schematic observation system. VoV1was fixed on a Ni2+-NTA-coated glass surface via His10tags in the A subunits and a bead was attached to a biotinylated Vo-c subunit. This VoV1had the TSSA mutation to suppress the ADPMg inhibition11. (b) Rotation observed at 2,000 fps at 40 μM ATP in the presence of 0.1% (w/v) Triton X-100. Horizontal lines are 30° apart. The time course is split into three and horizontally shifted (orange and green curves partially overlap). The record was divided into four coloured portions (black, magenta, orange and green) covering∼1 revolution and analysed as described inFigure 4. The angle 0, a start of a revolution on the vertical axis of the figure, was assigned to the red dot in each inset, chosen from the 12 orange spokes that fitted the dwells. The green line on the time courses shows 21-point (10 ms) median. Boxes enclosing trajectories measure 66×66 nm2. Histogram bin size is 3°. (c) Autocorrelation of the angular histogram: the continuous time courses over 1,500° were 21-point median filtered and then binned at 0.25° intervals without the correction for rotational drift. (d) The power spectrum ofc, the arrowhead showing a peak at (32°)−1. In Figure 4e,f , the average of all autocorrelations of individual angular histograms and its power spectrum, including other examples of ∼ 30° step rotation shown in Figure 5 and Supplementary Figures S2a,b is shown. The power spectrum in Figure 4f shows a peak at (32°) −1 . Figure 4: Well-resolved substeps in V o V 1 . ( a ) An expanded time course of the rotation of a 40-nm gold bead attached on a V o V 1 at 40 μM ATP, in the presence of 0.1% (w/v) Triton captured at 2,000 fps. Horizontal lines are 30° apart. The time course is split into three and horizontally shifted (magenta and orange curves partially overlap). To minimize the effect of small, gradual drift on the angle analysis, the record was divided into six coloured portions (black, magenta, orange, green, blue and purple) covering ∼ 1 revolution and analysed as follows. First, the bead trajectory in each portion (coloured square insets; grey points show raw data and black after 21-point median filtering of x and y time courses) was fitted with an ellipsoid (orange). Rotary angle was calculated by assuming the ellipsoid to be a projection of a circular orbit ( b ). The angle 0, a start of a revolution on the vertical axis of the figure, was assigned to the red dot in each inset, chosen from the 12 orange spokes that fitted the dwells. The green line on the time courses shows 41-point (20 ms) median. The histograms on the left axis represent logarithm of the number of data points per 2°. Red arrowheads, dwells that are clearly out of the 30° periodicity. Black arrowheads, excursions to a neighbouring (closed, forward; open, backward) dwell position for >20° and >20 ms. Boxes enclosing trajectories show a fixed 89×89 nm 2 area, such that drifts manifest as differences between insets. ( b ) Circular orbit (cyan) of a bead projected on the image plane (pink). Direction of observation is indicated by a green arrow. For the data in a , the angle θ ranged between 43° and 55°. ( c ) The autocorrelation of the angular histogram derived from a ; the continuous time course over 2,500° was 21-point median filtered and then binned at 0.25° intervals. For this analysis, we calculated the angular histogram without adjusting the angular origins of the six portions, that is, without correction for the rotational drift, to eliminate possible subjectivity. ( d ) The power spectrum of c , the arrowhead showing a peak at (27°) −1 . ( e ) The average of autocorrelations of individual angular histograms for Figures 4c , 5c and Supplementary Figures S2a,b . ( f ) The power spectrum of e , the arrowhead showing a peak at (32°) −1 . Full size image Figure 5: Substep rotation in upside up V o V 1 . ( a ) Schematic observation system. V o V 1 was fixed on a Ni 2+ -NTA-coated glass surface via His 10 tags in the A subunits and a bead was attached to a biotinylated V o -c subunit. This V o V 1 had the TSSA mutation to suppress the ADPMg inhibition [11] . ( b ) Rotation observed at 2,000 fps at 40 μM ATP in the presence of 0.1% (w/v) Triton X-100. Horizontal lines are 30° apart. The time course is split into three and horizontally shifted (orange and green curves partially overlap). The record was divided into four coloured portions (black, magenta, orange and green) covering ∼ 1 revolution and analysed as described in Figure 4 . The angle 0, a start of a revolution on the vertical axis of the figure, was assigned to the red dot in each inset, chosen from the 12 orange spokes that fitted the dwells. The green line on the time courses shows 21-point (10 ms) median. Boxes enclosing trajectories measure 66×66 nm 2 . Histogram bin size is 3°. ( c ) Autocorrelation of the angular histogram: the continuous time courses over 1,500° were 21-point median filtered and then binned at 0.25° intervals without the correction for rotational drift. ( d ) The power spectrum of c , the arrowhead showing a peak at (32°) −1 . Full size image In Figure 5 , in particular, V o V 1 was fixed upside up on a Ni 2+ -NTA-coated glass surface via His 10 tags in the A subunits and beads were attached with biotinylated V o -c subunit (see Fig. 5a ). The ∼ 30° steps are not the consequences of the upside down configuration ( Fig. 5b–d ). Taking into account the variations in the peak position in the individual power spectra, we conclude that substeps in V o V 1 rotation are characterized by an amplitude between 27°–32°. We noticed that some dwells were observed between two ∼ 30° dwell positions ( Fig. 4 , orange arrow heads). These may represent ATP-waiting dwells, because they were roughly 120° apart, taking the drift into account. If so, the ∼ 30° steps are not synchronous with ATP binding. This is not entirely unexpected, if the ∼ 30° steps arise from the stator–rotor interaction in the V o domain, whereas ATP binding takes place in V 1 . As mentioned above, ATP-waiting dwells in V o V 1 do not stand out even at low [ATP]. This suggests that the driving torque produced in the V 1 portion, the torque that can drive the DF rotor of V 1 over 120° in a matter of 0.25 ms or less, is sustained for many seconds while the V o rotor slowly proceeds over the bumps presented by the V o stator every ∼ 30°. An alternative, less likely scenario is that every ∼ 30° step is driven by ATP binding: because of friction in V o , V o V 1 works in a half-engaged clutch mode where 120° rotation in V 1 results in ∼ 30° rotation in V o . We also noticed that, during a long dwell, momentary excursions to a neighbouring dwell position took place in either direction, mostly forward. In Figure 4a and Supplementary Figure S2 , we indicate conspicuous excursions (amplitude >20° and duration >20 ms) with black arrowheads, counting 49 forward (closed arrowheads) and ten backward (open) ones in the total of 17 revolutions. The basically rectangular time courses seen in the expanded insets indicate metastable nature of the neighbouring dwell positions, consistent with bumps of structural origin as with the V o -c and V o -a interaction. We have characterized the ATP-driven rotation of both V 1 and V o V 1 under the conditions where the viscous drag between the probe and medium is negligible. For V 1 , the major results are that it pauses every 120° at all [ATP] ( Fig. 2 ), implying that the pauses occur at ATP-waiting angles, and that at least two reactions other than ATP-binding limit each dwell. No dwells at other positions are resolved, at the resolution of ∼ 0.1 ms, in contrast to F 1 that shows millisecond dwells at ∼ 80° past ATP-waiting angles. The previous study using a mutated V 1 and a slowly hydrolyzed ATP analogue suggested that hydrolysis in V 1 occurs at 0° (ATP-waiting angle), as opposed to the 80° hydrolysis in F 1 [15] , but absence of an 80° reaction(s) could not be demonstrated. In F 1 , another reaction, Pi release, takes place at ∼ 80°, contributing to the millisecond ∼ 80° dwells that are resolved even at saturating [ATP] if the temporal resolution is sufficiently high [15] , [16] . By contrast, the present results show that catalytic events in V 1 , at least those that take longer than a submillisecond, all occur at the ATP-binding position. At least two events other than ATP binding occur at this position, one likely to be ATP hydrolysis and the other phosphate or ADP release (or both combined). Together, it is safe to conclude that the canonical '80° and 40° scheme' for F 1 does not apply to V 1 . V o V 1 shows significantly different rotation behaviours from that of V 1 . V o V 1 rotated an order of magnitude slower. V o V 1 did not show clear 120° steps as observed in V 1 , and instead exhibited short pauses separated by ∼ 30°. We could not judge whether the [ATP] dependence of the rotation speed of V o V 1 follows simple Michaelis–Menten kinetics because of the large scatters in the data ( Fig. 1c ). At all [ATP], the rotary speed of V o V 1 was significantly lower than that of V 1 . The bumps introduced by the V o addition are high, such that passage has to wait for a rare thermal activation. The bumps also obscured ATP-waiting angles, although the angular histograms ( Fig. 3 , insets) indicate three broad peaks separated by ∼ 120°. Note that the ATP-waiting angles clearly observed in F 1 or V 1 represent the most stable orientation of the rotor in the ATP-waiting state. The rotor thermally fluctuates around this angle and actual ATP binding can take place at any point around the most stable angle [25] , [26] , [27] . In the presence of the V o bumps, the motor would wait for ATP on either side of a bump [16] , [28] , resulting in more than three ATP-waiting angles. The slow substep rotation of V o V 1 observed here is at odds with our previous observation with a duplex of 220-nm beads on the same upside down system (the A subunits were mutated to render the enzyme less prone to MgADP inhibition) [14] : the average rate of rotation was ∼ 10 r.p.s. at saturating [ATP], and the molecules basically showed 120° stepwise rotation at low [ATP]. Defective interaction in the V o domain could explain the discrepancy, although we are not sure if this was really the case. The ∼ 30° steps that we resolve relatively clearly in the presence of Triton are commensurate with the periodicity of the V o rotor ring in T. thermophilus V-ATPase [7] . It is highly likely that dwells result from specific interaction between a V o -c subunit in the ring and the V o -a subunit in the stator. When V o V 1 works as an ATP-driven proton pump in a membrane, proton translocation occurs at the interface between V o -c and V o -a. It is possible that protons were also translocated in our experiment with detergent-solubilized V o V 1 on a glass surface at one proton per ∼ 30° step. The momentary excursions to a neighbouring ∼ 30° position reinforce that the ∼ 30° bumps are of structural origin. Presumably, ATP hydrolysis reaction in V 1 domain sets up an energy slope that biases the thermal ride over bumps in the anticlockwise direction, and the elastic nature of the rotor [29] helps go over the bumps. Note that this view alone does not account for the strong tendency to rotate back to the original dwelling position after an excursion: the original position is somehow more stable than that of its neighbours. An obvious explanation would be the stable positions being next to an ATP-waiting angle, which must pose an energy valley until the next ATP binds. Indeed, starting angles of the excursions are grossly clustered at ∼ 120° intervals, supporting this interpretation. The 120° intervals, however, were not strictly observed and there were excursions from other angles. These are likely statistical exceptions, but might point to a remote possibility that the rotor–stator interaction is not static and each time it is reconfigured, possibly accompanying protonation/deprotonation, to make the new position stable; until that happens, the previous position remains more stable. Recently, Düser et al . [30] have reported stepwise c-ring rotation relative to the stator a subunits, equivalent to V o -a subunit of our V o V 1 , in E. coli F o F 1 during ATP synthesis using single-molecule fluorescence resonance energy transfer. They estimate the step size as ∼ 36°, which is consistent with the proposed c subunit stoichiometry of 10 in E. coli F o F 1 . In their experiment, protons, presumably each one of them, directly drive the rotation of the F o motor, whereas in our experiment the V o motor is passively driven by the V 1 motor and proton translocation would be the result and not the cause. The ∼ 30° steps we have observed indicate that passive interactions in the V o domain, possibly coupled to proton translocation, check and set the pace of ATP-driven rotation. Proteins The His-tagged V 1 (A (His−10/C28S/C508S)3 B (C264S)3 D (E48C/Q55C) F) was expressed in E. coli . After disruption of the cells by sonication, the his-tagged V 1 was purified by Ni2+-affinity column (Qiagen) and RESOURCE Q column (GE healthcare) [11] . The purified his-tagged V 1 was biotinylated at two cysteines using 6-[N-[2-(N-maleimide)ethyl]-N-piperazinylamide]hexyl- D -biotinamide (Dojindo). The V o V 1 for rotation assay was obtained by reconstitution of the V o containing a His 3 tag in each V o -c subunit and the Avi-Tagged V 1 [14] . The bound ADP in V 1 or V o V 1 was partially removed by successive EDTA–heat treatments [14] . Observation of rotation of 40-nm gold beads Streptavidin-coated 40-nm gold beads and Ni 2+ -NTA-coated cover glass were prepared [28] , [31] . A flow cell (5–10 μl) was made of two coverslips: a Ni 2+ -NTA-coated bottom one (24×36 mm 2 ) and an untreated top one (24×24 mm 2 ) separated by two spacers of 50 μm thickness. The biotinylated V 1 or Avitagged V o V 1 (1–5 nM) in buffer A (50 mM Hepes-KOH, pH8.0, 100 mM KCl, with 0.05% (w/v) DDM only for V o V 1 ) was applied to the flow cell and incubated for a few minutes. Unbound V 1 or V o V 1 was washed out with 20 μl of buffer A more than three times. Then, 20 μl of buffer A with 10 mg ml −1 BSA was infused to the flow cell and incubated for ∼ 30 s to prevent nonspecific binding. The BSA solution in the chamber was washed out with 20 μl of buffer A more than five times. Then, buffer A containing streptavidin-coated 40-nm beads (10 10 ∼ 10 11 particles per ml) were infused into the flow cell and incubated for a few min. Unbound gold beads were washed out with 20 μl of buffer A more than five times. After infusion of 80 μl of buffer A containing Mg-ATP at the indicated concentration, 2 mM MgCl 2 , 2.5 mM phosphoenol pyruvate and 0.5 mg ml −1 pyruvate kinase, bead rotation was observed at 23 °C by laser dark-field microscope [15] on an inverted microscope (Olympus IX70) with a stable microscope stage (KS-O, Chuukoshaseisakujo), with some modifications [28] (S. Furuike, unpublished): in place of the oblique laser-illumination [15] , the specimen was illuminated along the optical axis with parallel beam (diameter ∼ 10 μm, power <10 mW), by collimating a laser beam (Millennia IIs, Spectra Physics) with an objective placed just before the specimen. After the specimen was illuminated, the transmitted beam was let out through a pinhole at the centre of a mirror while the mirror deflected the scattered light to form a dark-field image of the beads. Images were captured with a high-speed CMOS camera (FASTCAM-DJV, Photron) at 250 to 8,000 frames per s as an 8-bit AVI file. Centroid of bead images was calculated [15] , [16] . How to cite this article: Furuike, S. et al . Resolving stepping rotation in Thermus thermophilus H + -ATPase/synthase with an essentially drag free probe. Nat. Commun. 2:233 doi: 10.1038/ncomms1215 (2011).